X-ray observation of a helium atom and placing a nitrogen atom inside He@C60and He@C70 Single crystal X-ray analysis has been used as a powerful method to determine the structure of molecules. However, crystallographic data containing helium has not been reported, owing to the difficulty in embedding helium into crystalline materials. Here we report the X-ray diffraction study of He@C 60 and the clear observation of a single helium atom inside C 60 . In addition, the close packing of a helium atom and a nitrogen atom inside fullerenes is realized using two stepwise insertion techniques, that is, molecular surgery to synthesize the fullerenes encapsulating a helium atom, followed by nitrogen radio-frequency plasma methods to generate the fullerenes encapsulating both helium and nitrogen atoms. Electron spin resonance analysis reveals that the encapsulated helium atom has a small but detectable influence on the electronic properties of the highly reactive nitrogen atom coexisting inside the fullerene, suggesting the potential usage of helium for controlling electronic properties of reactive species. The importance of helium is widely seen in its common use in helium balloons or respirator gas, as well as in its scientific use as a refrigerant for superconductive magnets and physical research at low temperature. Helium is well known as the smallest noble gas atom and it has refused to be directly observed by single crystal X-ray analysis, a powerful method to determine molecular structure. This is because neither helium nor a helium-incorporating material becomes crystalline solid under atmospheric pressure even in the vicinity of 0 K (ref. 1 ). Thus, it is crucial to embed a helium atom selectively into some crystalline material with a discrete structure if one wishes to observe it by X-ray analysis. Because the strength of the X-ray diffraction of single crystal X-ray analyses depends on the total number of electrons of all atoms existing in the unit cell, it is usually difficult to observe atoms with poor electron density, such as hydrogen, after structural refinements. In contrast, if a proper single crystal is available, a helium atom should be observable by the single X-ray analysis because a helium atom possesses two electrons in its 1s electronic shell which is isoelectronic with the lithium cation widely observed in the literature [2] . Fullerene C 60 is a good candidate to entrap a helium atom. Endohedral C 60 and C 70 encapsulating a helium atom, that is, 3 He@C 60 and 3 He@C 70 were first reported by Saunders et al . [3] in 1994 in which 3 He atom was forced into pristine C 60 and C 70 under drastic conditions, such as 650 °C under 3000, atm of helium gas [3] , [4] . However, the encapsulation level of the helium atom was quite low such as 0.15–0.4% (refs 5 , 6 ) because of the inefficiency of this physical method, although the inner 3 He atom is useful for the clarification of the internal magnetic field of fullerenes [5] . On the other hand, we have developed rational synthetic methodology [7] , [8] , [9] , [10] , [11] , [12] , [13] , [14] , [15] , so-called ‘molecular surgery’ [16] , and recently succeeded in the chemical syntheses of He@C 60 and He@C 70 with ca. 30% encapsulation levels in macroscopic scales. This method involves insertion of a helium atom into open-cage fullerene derivatives followed by restoration of the openings under mild conditions [14] . The encapsulation level of He@C 60 thus obtained was enhanced to 95% by purification with recycling high-performance liquid chromatography (HPLC) [14] . Here we report the single crystal X-ray observation of a helium atom inside C 60 . In addition, we also report the close contact of the helium atom with a nitrogen atom by placing a nitrogen atom inside He@C 60 and He@C 70 by the use of nitrogen radio-frequency (RF) plasma method [17] , [18] , [19] . Single crystal X-ray analysis of He@C 60 Although C 60 is a crystalline material, a C 60 cage is known to rotate even in the solid state [20] . To prevent such a rotational or orientational disorder in the single crystal, co-crystals of the He@C 60 and nickel(II) octaethylporphyrin (NiOEP) were prepared from the solution in o -xylene [15] , [21] . The X-ray diffraction data were collected using synchrotron radiation at 173 K at SPring-8. The least-square refinements gave the structure of He@C 60 ·(NiOEP) 2 without any disorders of the C 60 cage ( Supplementary Tables S1–S3 ). As shown in Fig. 1 , the encapsulated helium atom was unambiguously observed at the centre of the C 60 cage with 100% occupation level, probably owing to the enrichment during crystallization. It should be mentioned that the position of the helium is similar to that of krypton reported by the X-ray diffraction data of (Kr@C 60 /C 60 )·(NiOEP)·2C 6 H 6 , with the occupation level of krypton being only 9% ( [21] ). The relatively larger ellipsoid of the helium implies its translational motion at this temperature because there remains small space for the encapsulated helium atom inside C 60 (estimated diameter of the hollow space is ca. 3.7 Å and the van der Waals diameter of helium is 2.80 Å (ref. 22 )). 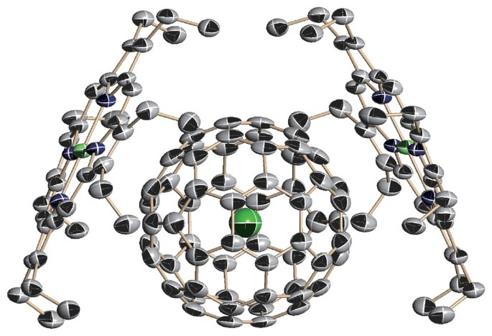Figure 1: X-ray crystal structure of He@C60·(NiOEP)2. Thermal ellipsoids at the 50% probability level and hydrogen atoms are omitted for clarity. NiOEP, nickel(II) octaethylporphyrin. Figure 1: X-ray crystal structure of He@C 60 ·(NiOEP) 2 . Thermal ellipsoids at the 50% probability level and hydrogen atoms are omitted for clarity. NiOEP, nickel(II) octaethylporphyrin. Full size image Insertion of a nitrogen atom to He@C 70 and He@C 60 After confirming the existence of one helium atom inside C 60 , we wondered about the capability of this complex to further accommodate an additional guest species. It seemed intriguing to see if so-believed ‘inert’ helium could affect the properties of a neighbour atom in tightly confined space inside He@C 60 or He@C 70 . For this purpose, a nitrogen atom was selected as the guest. It is reported that a sharp triplet electron spin resonance (ESR) signal is observed for the reaction products of C 60 and C 70 with a nitrogen atom source (see below), indicating the generation of N@C 60 and N@C 70 ( [23] , [24] , [25] , [26] ). The inner nitrogen atom of these endofullerenes retains its electron spin of 3/2 without any covalent bond formation with carbons of the C 60 or C 70 cage. These products are believed to be endohedral fullerenes, which are promising materials for quantum computers [27] , [28] . Insertion of a nitrogen atom into He@C 70 ( ca. 30% encapsulation level), whose inner space (estimated long axis diameter is ca. 4.7 Å) is larger than that of He@C 60 , was conducted under the nitrogen RF plasma conditions [17] , [18] , [19] . As shown in Fig. 2a (also see Supplementary Fig. S1 ), the ESR spectrum of the resulting material showed a new triplet signal in addition to a larger triplet corresponding to N@C 70 with the hyperfine coupling constant (hfcc) of 5.38 Gauss as reported [27] . In spite of a partial overlap with the known triplet corresponding to N@C 70 , a simulated spectrum revealed the presence of a new species with the hfcc of 5.59 Gauss. This result is most reasonably interpreted by the generation of C 70 , encapsulating both helium and nitrogen atoms, that is, HeN@C 70 . The existence of HeN@C 70 was also confirmed by mass spectrometry of the enriched sample prepared by repeated recycling HPLC ( Supplementary Fig. S2 ). Moreover, though the inner space of He@C 60 seemed too small to accommodate a nitrogen atom as an additional guest, similarly overlapped ESR signals were obtained when He@C 60 ( ca. 30% encapsulation level) was used for the nitrogen insertion ( Fig. 2b ), indicating the generation of HeN@C 60 . The hfcc of HeN@C 60 (5.99 Gauss) is slightly larger than that of N@C 60 (5.67 Gauss). The ratio of the integrated peak areas of HeN@C 60 /N@C 60 (1/9) was lower than that of HeN@C 70 /N@C 70 (3/7) at room temperature. This difference implies that it is easier for a nitrogen atom to access to the larger inner space of He@C 70 than that of He@C 60 . 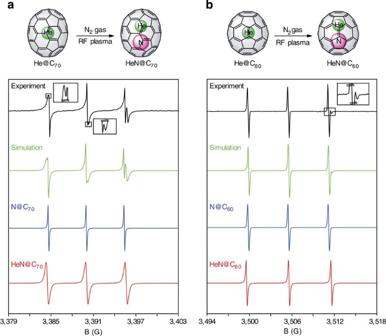Figure 2: Generation of the C70and C60incorporating a helium atom and a nitrogen atom. (a) Experimental ESR spectrum ofHeN@C70and N@C70in CS2at 220 K (black line), and simulated spectra of the mixture (green line), N@C70(blue line) andHeN@C70(red line), respectively. (b) Experimental ESR spectrum ofHeN@C60and N@C60in CS2at room temperature (black line), and simulated spectra of the mixture (green line), N@C60(blue line) andHeN@C60(red line), respectively. Figure 2: Generation of the C 70 and C 60 incorporating a helium atom and a nitrogen atom. ( a ) Experimental ESR spectrum of HeN@C 70 and N@C 70 in CS 2 at 220 K (black line), and simulated spectra of the mixture (green line), N@C 70 (blue line) and HeN@C 70 (red line), respectively. ( b ) Experimental ESR spectrum of HeN@C 60 and N@C 60 in CS 2 at room temperature (black line), and simulated spectra of the mixture (green line), N@C 60 (blue line) and HeN@C 60 (red line), respectively. Full size image The inner nitrogen atoms of HeN@C 60 and HeN@C 70 still retain the electron spin state of 3/2, in spite of the existence of the tightly packed helium atom, showing the entire inertness of helium. However, the line widths of three signals for HeN@C 60 and HeN@C 70 are clearly broadened compared with those for N@C 60 and N@C 70 . This is because placing a helium atom inside N@C 60 and N@C 70 causes lower symmetry of the resulting HeN@C 60 and HeN@C 70 compared with high symmetry of the starting materials. Such lower symmetry of the molecules breaks the degeneracy of the three 2p orbitals of the inner nitrogen atom, giving rise to appearance of the broad signals in which possible fine structures are about to appear. This is consistent with the reported observations on N@C 60 derivatives with exohedral functionalizations [29] , [30] . To gain insight into the structures and properties of HeN@C 60 , theoretical consideration was essential. The structures of the related molecules were fully optimized at the M06-2X [31] method using basis sets of 6-31G(d) [32] for C and 6-311+G(2df) [33] for He and N atoms [34] ( Supplementary Tables S4–S6 ). It was shown that the encapsulation of both helium and nitrogen atoms into C 60 is exothermic by −7.1 kcal mol −1 after correction of basis set superposition error. This stabilization energy of HeN@C 60 is lower than that of N@C 60 (–23.4 kcal mol −1 ), but higher than that of He@C 60 (–3.2 kcal mol −1 ), indicating that the coexistence of the two atoms in a small space inside C 60 could be reasonable. It is considered that these atoms are packed tightly inside the C 60 cage because the distance between the helium and the nitrogen atoms (2.07 Å) was obviously shorter than that at the most stable position (3.75 Å) calculated at the CCSD(T)/6-311+G(2df) level of theory. Using the optimized structures at the M06-2X method, the hfcc values were studied by the single-point calculations at MP2 [35] method using basis sets of 6-31G(d) for C and 6-311++G(3df,3pd) for He and N atoms. The calculated hfcc values were found to highly depend on the basis sets. Among the tested basis sets, the use of 6-311++G(3df,3pd) gave the acceptable results for N@C 60 as a benchmark compound; the calculated and experimental hfcc values are 5.44 and 5.67 Gauss, respectively. As shown in Fig. 3a , the calculated hfcc values reproduced the experimental tendency that the smaller space for a nitrogen atom results in the larger hfcc (5.57 Gauss for HeN@C 60 ), most probably owing to the increased s electron density on the nucleus of the nitrogen. To clarify the contributing factors of this phenomenon, the He atom in the optimized structure of HeN@C 60 was removed, and the hfcc of the remaining N atom located at off-centre inside C 60 was calculated as the hypothetical molecule to afford the larger hfcc value of 5.80 Gauss ( Fig. 3a : HeN@C 60 –He). These results indicated that the hfcc of the nitrogen is larger, as the distance between the N atom and the fullerene cage becomes shorter. On the contrary, the hfcc value of a nitrogen atom with a neighbouring helium atom in a distance of 2.07 Å (3.52 Gauss) was smaller than that with a helium atom at the optimized distance of 3.75 Å (3.66 Gauss) or without a helium atom (3.69 Gauss) ( Fig. 3b ). These results showed that the hfcc values decrease as the helium atom gets closer to the nitrogen atom. Thus, the experimentally observed increase in hfcc value for HeN@C 60 compared with that of N@C 60 is rationalized in terms of the compensation of the increase by the C 60 cage and the decrease by the neighbouring helium atom. 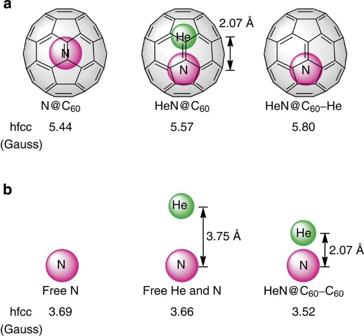Figure 3: Calculated hfccs of nitrogen atoms at the MP2 level. (a) The hfccs of N@C60,HeN@C60andHeN@C60–He (the helium atom being removed from the optimized structure ofHeN@C60). (b) The hfccs of a free nitrogen atom and the nitrogen atoms with a neighbouring helium atom at the distance of 3.75 Å (optimized distance) and 2.07 Å (extracted distance fromHeN@C60). Figure 3: Calculated hfccs of nitrogen atoms at the MP2 level. ( a ) The hfccs of N@C 60 , HeN@C 60 and HeN@C 60 –He (the helium atom being removed from the optimized structure of HeN@C 60 ). ( b ) The hfccs of a free nitrogen atom and the nitrogen atoms with a neighbouring helium atom at the distance of 3.75 Å (optimized distance) and 2.07 Å (extracted distance from HeN@C 60 ). Full size image To obtain more information on the inner encapsulated atoms of helium and nitrogen, the Atoms-in-Molecules (AIM) analysis [36] was carried out at the MP2 level with the optimized structure at the M06-2X method described above, using the AIM 2000 package program (version 2.0). In the AIM analysis, if the bond path through the bond critical point (BCP) connects two atoms, it is defined to be an interaction existing between these atoms. As shown in Fig. 4 , there is a bond path between the He atom and the N atom. There are also three He–C and four N–C bond paths in the C 60 cage ( Fig. 4a ). These results imply that not only the C 60 cage but also the He atom interact with the N atom. By the analysis at the BCP ( Supplementary Fig. S3 ) [36] , the inner N atom is not covalently bound with the He atom nor C 60 cage. Comprehensively, the He atom and the N atom interact with each other only through a van der Waals interaction inside the C 60 cage, whose situation is similar to that of He 2 @C 60 (ref. 37 ). 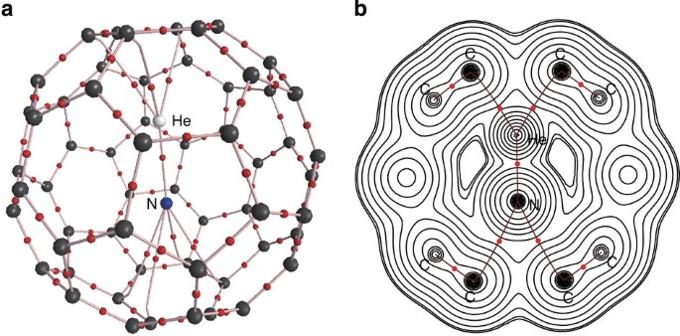Figure 4: AIM analysis ofHeN@C60at the MP2 level. (a) Molecular depiction with displaying BCPs in red. (b) Cross-section contour map of electron density with bond paths in brown and BCPs in red. The contours [ea0–3] are at 2l(l=±8, ±7,..., 0), and 0.0047 (heavy line). Figure 4: AIM analysis of HeN@C 60 at the MP2 level. ( a ) Molecular depiction with displaying BCPs in red. ( b ) Cross-section contour map of electron density with bond paths in brown and BCPs in red. The contours [ ea 0 –3 ] are at 2 l ( l =±8, ±7,..., 0), and 0.0047 (heavy line). Full size image The present result clearly showed that a single atom of helium in C 60 is observable by means of single crystal X-ray analyses. Thus, the element of helium newly joined the libraries of X-ray crystallographic study [38] . The encapsulated helium was confirmed to be located at the centre inside the C 60 . In addition, the stepwise insertion of different atoms into fullerenes was achieved by the combined ‘molecular surgery’ and ‘nitrogen RF plasma’ methods. Even highly reactive nitrogen atom was found to coexist with a helium atom in a small space inside fullerenes. The ESR signals of the nitrogen atom were influenced by the helium coexisting in the same fullerene cages. Thus, these results are considered to be pieces of evidence for encapsulation of a nitrogen atom inside fullerenes. This technique is expected to create a variety of endohedral fullerenes, encapsulating heterogeneous atoms in the near future. General He@C 60 and He@C 70 were synthesized by following our previous report [14] . ESR spectra were measured by Bruker EMX and EMX plus spectrometers. The temperature was controlled with an Oxford ESR900 helium flow-type cryostat and an Oxford ITC503 temperature controller for the EMX plus. Simulation of the spectra was carried out on a WinSim program [39] . The atmospheric pressure chemical ionization mass spectrum was recorded on a Bruker micrOTOF-QII. Single-crystal X-ray analysis of He@C 60 ·(NiOEP) 2 Single-crystal X-ray data were collected on a BL38B1 beamline in SPring-8 with the approval of the Japan Synchrotron Radiation Research Institute with a diffractometer equipped with an ADSC Quantum 315 CCD (charge-coupled device) detector. The collected diffraction data were processed with the HKL2000 software program. The structure solutions were obtained by direct method using the SHELXS-97 program [40] and refined using the SHELXL-97 program [40] . Experimental details for generation of HeN@C 60 or HeN@C 70 HeN@C 60 or HeN@C 70 was generated by a nitrogen RF plasma method [17] . He-encapsulating fullerene, He@C 60 or He@C 70 , (~9 mg, ca. 30% encapsulation level) was put in a molybdenum boat and placed into the instrument. Under the reduced pressure of nitrogen gas (30 Pa), the material containing N-encapsulating fullerene was generated by sublimation through resistive heating in nitrogen plasma. After cooling to room temperature, the deposit (~3 mg) was dissolved in CS 2 , followed by filtration and evaporation of the solvent. The resulting material was dissolved in toluene and subjected to recycling HPLC equipped with the Cosmosil Buckyprep column (250 mm length, 20 mm inner diameter; mobile phase, toluene) for further purification. The major fraction was collected and evaporated. The residue was dissolved in CS 2 and placed in an ESR tube, which was connected to a vacuum line. The solution was degassed by three freeze-pump thaw cycles under reduced pressure, and then sealed. Enrichment of HeN@C 70 After sublimation of He@C 70 /C 70 (3/7) through resistive heating in nitrogen plasma, the resulting deposit (~3 mg) was subjected to the recycle HPLC equipped with the Cosmosil Buckyprep columns (two directly connected columns; 250 mm length, 20 mm inner diameter; mobile phase, toluene; 25 °C; flow rate was 8.0 ml min –1 ). The retention time of HeN@C 70 was close to that of N@C 70 ( [25] ). After two recycling, the latter portion of main peak was evaporated and further subjected to the same HPLC to enrich HeN@C 70 . The existence of HeN@C 70 and N@C 70 was monitored by the ESR spectra. After repeating this procedure five times, the resulting mixture in toluene solution (100 μl) was subjected to a Bruker micrOTOF-QII to give the mass spectrum shown in Supplementary Fig. S2 . Theoretical methods Geometries were fully optimized with hybrid density functional theory at the M06-2X ( [31] ) level. The 6-31G(d) basis set [32] was used for C, whereas the 6-311+G(2df) basis set [33] was used for He and N. To calculate the hfccs, the M06-2X optimization was followed by single-point MP2 (second-order Møller–Plesset perturbation theory) [35] calculations using 6-311++G(3df, 3pd) basis set for He and N, and 6-31G (d) basis set for C. Calculations were carried out using the GAUSSIAN 09 program [34] . Accession codes: The X-ray crystallographic coordinates for the structure reported in this Article has been deposited at the Cambridge Crystallographic Data Centre (CCDC), under deposition number CCDC 921390. These data can be obtained free of charge from The Cambridge Crystallographic Data Centre via www.ccdc.cam.ac.uk/data_request/cif . How to cite this article: Morinaka, Y. et al . X-ray observation of a helium atom and placing a nitrogen atom inside He@C 60 and He@C 70 . Nat . Commun . 4:1554 doi: 10.1038/ncomms2574 (2013).